X-ray micro-beam characterization of lattice rotations and distortions due to an individual dislocation Understanding and controlling the behaviour of dislocations is crucial for a wide range of applications, from nano-electronics and solar cells to structural engineering alloys. Quantitative X-ray diffraction measurements of the strain fields due to individual dislocations, particularly in the bulk, however, have thus far remained elusive. Here we report the first characterization of a single dislocation in a freestanding GaAs/In 0.2 Ga 0.8 As/GaAs membrane by synchrotron X-ray micro-beam Laue diffraction. Our experimental X-ray data agrees closely with textbook anisotropic elasticity solutions for dislocations, providing one of few experimental validations of this fundamental theory. On the basis of the experimental uncertainty in our measurements, we predict the X-ray beam size required for three-dimensional measurements of lattice strains and rotations due to individual dislocations in the material bulk. These findings have important implications for the in situ study of dislocation structure formation, self-organization and evolution in the bulk. Dislocations are crystallographic defects that allow the minimization of strain energy through the localization of crystal lattice distortion [1] . Their behaviour is of fundamental importance for the performance of thermoelectric devices [2] , nano-electronics [3] , [4] and solar cells [5] , [6] . In structural engineering alloys, used for high-performance aerospace applications, dislocation-mediated slip is one of the main deformation mechanisms [7] . To optimize material strength and resistance to failure, careful management of dislocation structures and their evolution is essential [8] , [9] . Transmission electron microscopy (TEM) revolutionized materials science through its ability to directly image individual dislocations [10] . However, it is limited by the need for thin, electron-transparent samples. These can be slices extracted ‘post mortem’ from the bulk or nano-sized samples deformed in situ . The former do not allow dynamic studies and in the latter behaviour may not be representative of the bulk due to size effects [11] . X-rays provide an alternative means of characterizing dislocations in the bulk without the need for sectioning. X-ray topography, which relies on the extinction contrast formed when the crystal lattice moves out of the Bragg condition, allows bulk single dislocation imaging [12] . However, it is confined to samples with small lattice rotations and low dislocation densities, and does not provide direct quantitative information, greatly limiting its range of applications. Synchrotron X-ray micro-beam Laue diffraction (μ-Laue), on the other hand, is perfectly suited to the mapping of polycrystalline samples and the study of steep orientation gradients [13] , [14] . It uses a focussed, polychromatic X-ray beam to probe submicron-sized scattering volumes. Provided the local crystal size is larger than the X-ray beam, a single-crystal Laue diffraction pattern is recorded. Lattice orientation and strain in the sampling volume are determined directly by fitting of the diffraction peak positions [15] , [16] , [17] . From streaking of Laue peaks and lattice orientation changes, the density of geometrically necessary dislocations can be inferred [18] , [19] . Using μ-Laue diffraction techniques [20] , the self-organized cell/wall structures formed by groups of dislocations in face-centred cubic single crystals [21] , as well as dislocation boundaries in epitaxial GaN films [22] , have been previously studied. An alternative technique, Bragg coherent diffractive imaging (BCDI), uses a coherent monochromatic X-ray beam to capture a three-dimensional (3D), ‘oversampled’ reciprocal space map of submicron, single crystalline samples [23] . Phase retrieval algorithms are employed to invert the reciprocal space map and reconstruct the complex electron density in the sample. Using this approach, 3D strain imaging has been successfully demonstrated in weakly strained objects [24] , [25] , [26] . The reconstruction of highly strained objects, such as dislocations, is far more challenging. Approaches to this problem have generally relied on a priori sample information [27] or model matching of diffraction patterns [28] . Recently some progress with single dislocation imaging has been made using Bragg ptychography, an extension of BCDI in which data from multiple overlapping scattering volumes is used in image reconstruction [29] . However, direct quantification, via X-ray diffraction, of the lattice rotations and strain fields associated with an individual dislocation has thus far remained elusive. In this paper, we demonstrate quantitative measurements of the lattice distortions due to an individual dislocation using μ-Laue diffraction. Specifically, we measure the lattice rotations and strain fields associated with a single misfit dislocation in a free-standing GaAs/In 0.2 Ga 0.8 As/GaAs membrane. This material has intrinsic scientific importance as a key ingredient in integrated circuits, light-emitting diodes and solar cells [30] , [31] . A thin membrane sample is chosen in order to allow a direct comparison with TEM. However, as our calculations demonstrate, there is no practical limitation on making these measurements in bulk materials, provided a sufficiently small polychromatic beam is available. Sample description and TEM measurements The sample consisted of a 60 nm GaAs/9.5 nm In 0.2 Ga 0.8 As/60 nm GaAs free-standing membrane manufactured by molecular beam epitaxy and ‘lift-off’ [32] . X-ray reflectance and BCDI were used to confirm the layer thicknesses. Lattice mismatch between GaAs and In 0.2 Ga 0.8 As layers gives rise to 60° misfit dislocations at their interface (schematically shown in Fig. 1a ). These dislocations, aligned along the <II0> directions, are several tens of microns long and form grids of parallel dislocations [32] . Splitting of the 60° misfit segments into partial dislocations has been observed [33] ; however, the separation between partials is much smaller than the present spatial resolution and hence the effects of dissociation can be treated as negligible. 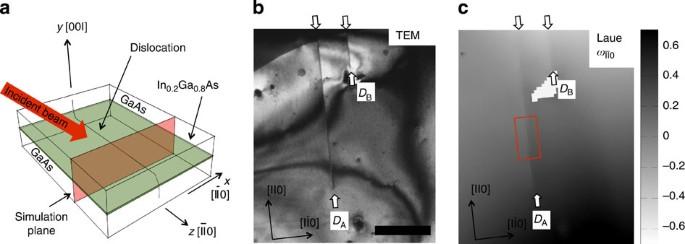Figure 1: Sample layout. (a) Schematic of the free-standing GaAs/In0.2Ga0.8As/GaAs membrane showing principal crystallographic directions, a misfit dislocation, the In0.2Ga0.8As layer (green), the simulation plane (red) and the incident X-ray beam. (b) Brightfield TEM of the sample showing two misfit dislocations,DAandDB. (c) Map of lattice rotation,ωĪĪ0, recorded using micro-beam Laue diffraction. Superimposed is a red box indicating the measurement region of the data shown inFig. 3. The scale bar inbrepresents a length of 10 μm andbandcare shown on the same scale. The colour bar incshows angular misorientation in degrees. Figure 1: Sample layout. ( a ) Schematic of the free-standing GaAs/In 0.2 Ga 0.8 As/GaAs membrane showing principal crystallographic directions, a misfit dislocation, the In 0.2 Ga 0.8 As layer (green), the simulation plane (red) and the incident X-ray beam. ( b ) Brightfield TEM of the sample showing two misfit dislocations, D A and D B . ( c ) Map of lattice rotation, ω ĪĪ0 , recorded using micro-beam Laue diffraction. Superimposed is a red box indicating the measurement region of the data shown in Fig. 3 . The scale bar in b represents a length of 10 μm and b and c are shown on the same scale. The colour bar in c shows angular misorientation in degrees. Full size image Figure 1b shows a bright field TEM image of the sample recorded with a JEOL 2010 F TEM operated at 200 kV. Two isolated misfit dislocations (labelled as D A and D B ) are clearly visible owing to diffraction contrast [10] . Some broader fringes are present owing to larger scale curvature of the membrane introduced during the ‘lift-off’ procedure. X-ray diffraction measurements μ-Laue diffraction measurements were made at beamline 34-ID-E at the Advanced Photon Source, Argonne National Lab, Illinois, USA [34] . A polychromatic X-ray beam (7–30 keV) focussed to a near Lorentzian-shaped probe spot with full width at half maximum (FWHM) of 0.6 μm vertically and 0.4 μm horizontally was used to illuminate the sample (see Methods section and Supplementary Fig. S1 ). From the Laue diffraction patterns, lattice rotations and strains were computed with respect to a nominally strain-free reference, thus removing systematic offsets. Figure 1c shows a μ-Laue map of lattice rotation, ω ĪĪ0 , about the [ĪĪ0] axis for the area imaged by TEM in Fig. 1b . A clear step change in lattice orientation due to dislocations D A and D B is visible. Both dislocations can be unambiguously identified. Laue patterns near the end of dislocation D B could not be indexed owing to poor pattern quality in this area, most likely as a result of sample contamination. To study lattice rotations and strains in detail, line profiles containing eight measurement points, evenly spaced in 0.5 μm intervals in the direction perpendicular to the line of dislocation D A , were considered. Overall 16 lines, positioned at 0.5 μm increments along the D A dislocation line in the [ĪĪ0] direction, were measured. This approach allowed for some imperfections in the alignment of TEM images and optical microscopy used to position the X-ray measurements. The corresponding measurement region is shown as a red box in Fig. 1c . The average of the line profiles at each point indicates the value of lattice rotation and strain, whereas their standard deviation captures the experimental uncertainty (see Fig. 3 and Supplementary Note 1 ). The measurement location of the line profiles was chosen to be remote from the ends of dislocations D A and D B , so that a comparison with the solution for an infinitely long 2D dislocation could be made. Elastic calculations of dislocation strain fields The expected lattice rotations and strains for an infinitely long 2D dislocation in a thin membrane were modelled by superimposing 2D plane strain anisotropic elasticity solutions for dislocations in an infinite medium [1] and a finite element calculation to solve the boundary value problem [35] (see Supplementary Figs S2 and S3 ). The misfit dislocation was assumed to lie in the mid-plane of the membrane, the presence of the InGaAs layer was neglected and GaAs was assumed to be anisotropically elastic with cubic symmetry [36] , [37] . 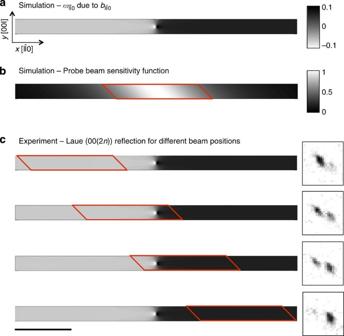Figure 2:ωorientation change. (a) Computed map of lattice rotationωabout the [ĪĪ0] axis due to the in-plane edge dislocation component with burgers vectorb=1.998 Å. This map corresponds to a section through the membrane, as illustrated inFig. 1a. The colour bar shows angular misorientation in degrees. (b) Plot of the normalized probe sensitivity function used to calculate the expected deviatoric strain profiles. The superimposed red parallelogram indicates the probe FWHM. (c) Raw images of the (00(2n)) Laue reflection for different probe centre positions with respect to the dislocation line. In each case, the region illuminated by the probe beam is illustrated by a red parallelogram, showing the beam’s FWHM, superimposed on a calculated plot ofωlattice rotation due tob(as in parta). The scale bar represents 500 nm and applies to all calculated maps ina,bandc. Figure 2a shows a map of the ω ĪĪ0 lattice rotation, calculated on the simulation plane shown in Fig. 1a , due to the edge component of the misfit dislocation with burgers vector in the membrane plane ( b IĪ0 =1.998 Å). A sharp change in ω ĪĪ0 lattice orientation (~0.1°), comparable to Fig. 1c , is evident at the dislocation line. The origin of this orientation change is similar to that in a tilt boundary [38] . Provided the dislocation is aligned perpendicular to the incident beam direction and the diffraction detector normal direction, as shown in Supplementary Fig. S1 , the lattice rotation of ~0.1° is sufficient to cause complete splitting of the Laue diffraction peaks as the probe beam (simulation shown in Fig. 2b ) approaches the dislocation line. This is illustrated by (00(2 n )) GaAs reflections recorded at different probe positions relative to the dislocation line ( Fig. 2c ). Owing to this splitting, the diffraction signals originating from either side of the dislocation line can be treated separately, provided a sufficiently small fitting window is used for every diffraction peak (here 7 × 7 pixels). This approach reduces strain averaging due to the probe size and yields a significant increase of the measurable strain. Figure 2: ω orientation change. ( a ) Computed map of lattice rotation ω about the [ĪĪ0] axis due to the in-plane edge dislocation component with burgers vector b =1.998 Å. This map corresponds to a section through the membrane, as illustrated in Fig. 1a . The colour bar shows angular misorientation in degrees. ( b ) Plot of the normalized probe sensitivity function used to calculate the expected deviatoric strain profiles. The superimposed red parallelogram indicates the probe FWHM. ( c ) Raw images of the (00(2n)) Laue reflection for different probe centre positions with respect to the dislocation line. In each case, the region illuminated by the probe beam is illustrated by a red parallelogram, showing the beam’s FWHM, superimposed on a calculated plot of ω lattice rotation due to b (as in part a ). The scale bar represents 500 nm and applies to all calculated maps in a , b and c . Full size image To model the elastic strain profiles expected in the Laue measurement, the deviatoric elastic strain field ε * ( x , y ) was calculated for the misfit dislocation in the membrane, where x corresponds to the [IĪ0], y to the [00I] and z to the [ĪĪ0] direction. The deviatoric strain field, as well as the associated stress and lattice rotation fields are shown in Supplementary Figs S4–S6 , respectively. Deviatoric strain is of interest since Laue diffraction without additional monochromatic measurements provides access to unit cell distortion only [39] . The ε * ( x , y ) field was convolved with a probe sensitivity function p ( x , y ) that captures the Lorentzian shape of the incident beam and accounts for finite attenuation length (see Fig. 2b and Supplementary Fig. S7 ). Diffraction from either side of the dislocation was treated separately, as in the experimental analysis. The expected lattice rotations were computed in the same manner. The resulting calculated line profiles for the six strain components and three lattice rotations are shown in Fig. 3 . Further details of these simulations are provided in Supplementary Notes 2 and 3 . 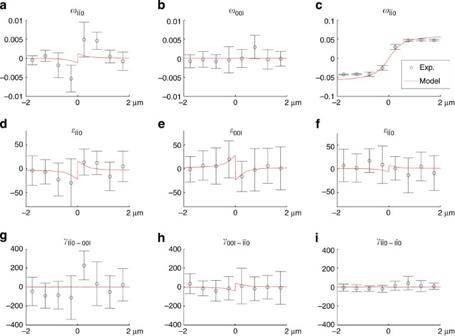Figure 3: Experimental and calculated lattice strain and rotation profiles. (a–c) Lattice rotations about the [IĪ0], [00I] and [ĪĪ0] axes, respectively, in degrees. (d–f) Direct elastic strains in the [IĪ0], [00I] and [ĪĪ0] directions, respectively, in units of 10−6. (g–i) Shear strains in the (ĪĪ0), (IĪ0) and (00I) planes, respectively, in units of 10−6. Measured and predicted profiles are plotted as a function of distance from the dislocation core along the samplex-axis, that is, the [IĪ0] direction. Figure 3: Experimental and calculated lattice strain and rotation profiles. ( a – c ) Lattice rotations about the [IĪ0], [00I] and [ĪĪ0] axes, respectively, in degrees. ( d – f ) Direct elastic strains in the [IĪ0], [00I] and [ĪĪ0] directions, respectively, in units of 10 −6 . ( g – i ) Shear strains in the (ĪĪ0), (IĪ0) and (00I) planes, respectively, in units of 10 −6 . Measured and predicted profiles are plotted as a function of distance from the dislocation core along the sample x -axis, that is, the [IĪ0] direction. Full size image The measured lattice rotation profiles ( Fig. 3a–c ) agree with our predictions. This stands as one of few direct experimental verifications of elasticity solutions for individual dislocations [40] , [41] , [42] . In the ω IĪ0 profile ( Fig. 3a ), the measured values are somewhat larger than the predicted ones. For the ω 00I rotation ( Fig. 3b ), both experimental and predicted values are zero as expected. The most prominent lattice rotation is observed for ω ĪĪ0 ( Fig. 3c ). This is due to the edge dislocation component with burgers vector b IĪ0 =1.998 Å, that causes a macroscopic fold in the membrane ( Fig. 2a ). The experimental profile shows a smaller change in lattice orientation across the dislocation line than predicted. A possible explanation is provided by macroscopic tension on the membrane due to remote constraint, which would act to reduce the orientation change. The direct elastic strains show a sign change in both the ε IĪ0 ( Fig. 3d ) and the ε 00I ( Fig. 3e ) components as the dislocation line is crossed. In particular, the measured ε 00I component follows the predicted profile closely. The predicted strain variation of the ε ĪĪ0 component ( Fig. 3f ) is smaller and cannot be clearly identified in the experimental data. The average strain uncertainty for the direct strains ε IĪ0 , ε 00I and ε ĪĪ0 is±33 × 10 −6 . This agrees well with previous estimates [16] , [17] . Interestingly the uncertainty of the shear strains γ IĪ0–00I and γ 00I–ĪĪ0 (±150 × 10 −6 ) ( Fig. 3g,h , respectively) is much larger than that of the γ ĪĪ0–IĪ0 component (±45 × 10 −6 ) ( Fig. 3i ) and the direct strains. This effect is due to the limited coverage of reciprocal space by the detector and is also prominently observed in calibration measurements of a Germanium wafer sample (see Supplementary Note 1 ). Because of the larger shear strain uncertainty the expected variation of the γ 00I–ĪĪ0 component cannot be seen in the experimental data. Simulations in which the elastic anisotropy of GaAs was neglected yielded predicted strain and rotation profiles similar to those found from elastically anisotropic calculations. The differences between isotropic and anisotropic models are small compared with the experimental uncertainty of the present measurements (see Supplementary Note 4 and Supplementary Figs S8–S11 ). To estimate the spatial resolution required to image individual dislocations in the bulk, a model of the misfit dislocation embedded in an infinite, anisotropic elastic medium was established (see Supplementary Fig. S12 ). Differential aperture X-ray microscopy (DAXM) allows depth resolution in μ-Laue measurements comparable to the incident beam size [20] . Hence we assumed a probe sensitivity function p ( x,y,z ) with the same FWHM and Lorentzian profile in all spatial directions. The deviatoric strain maps that would be measured with different size probes were computed by convolving the calculated deviatoric strain field with the probe sensitivity function (see Supplementary Note 5 and Supplementary Fig. S13 ). 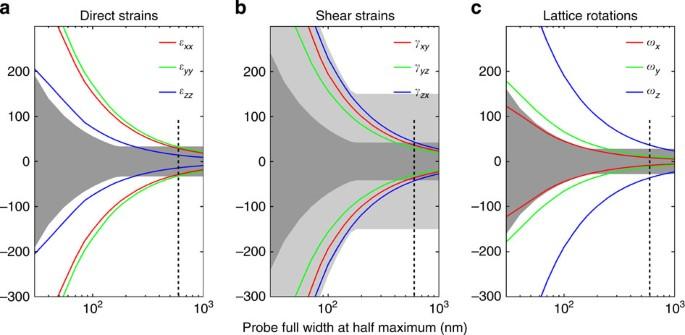Figure 4: Strain and lattice rotation. Estimated minimum and maximum strain and lattice rotation values for a misfit dislocation buried in the bulk. The vertical axes show direct strains (a) and shear strains (b) in units of micro strain (10−6), and lattice rotations (c) in degrees. The horizontal axes show the probe FWHM in nm. In the strain and lattice rotation subscripts,xcorresponds to the [IĪ0],yto the [00I] andzto the [ĪĪ0] direction. Superimposed in grey are the estimated experimental uncertainties. Inb, the light grey area shows the anticipated uncertainty associated with theγxyandγyz(that is,γ–00Iandγ00I–) shear strain components, whereas the dark grey area shows the uncertainty associated with theγzx(that is,γ–) component. The vertical dashed lines indicate the X-ray probe size used for the experiments reported here. Figure 4 shows a plot of the anticipated maximum and minimum signal for the direct strains ( Fig. 4a ), shear strains ( Fig. 4b ) and lattice rotations ( Fig. 4c ) as a function of probe FWHM. Superimposed on these plots are also estimates of the anticipated experimental uncertainties based on the probe beam divergence (see Supplementary Table S1 ) and the measured strain and rotation uncertainties (see Supplementary Table S2 and Supplementary Note 5 ). Clearly for the present probe FWHM of 600 nm, the signal due to a single dislocation in the material bulk would be smaller than the measurement uncertainty. As the beam size is reduced the expected signal becomes more prominent, and should be unambiguously measurable with beam sizes smaller than 200 nm. Interestingly the large uncertainties associated with the γ IĪ0–00I and γ 00I–ĪĪ0 shear strain components preclude the measurement of these strain components irrespective of beam size. Instead a more complete coverage of reciprocal space using larger or multiple area detectors is required to reduce the uncertainty associated with these strain components. Simulations using a 3D Gaussian probe sensitivity function showed a small increase in the expected signal, but overall the effect of the exact beam shape appears to be small. One might also expect a loss of DAXM depth resolution due to increasing beam divergence as the diffraction-limited beam size is reduced. However, for beam sizes >25 nm and measurement depths of a few microns, this is likely to be a minor effect. Sub 200 nm achromatic focussing has already been demonstrated [43] , indeed the record for the smallest hard X-ray focal spot size obtained using achromatic Kirkpatrick–Baez mirrors is currently 25 nm [44] . Incorporating these focussing optics into μ-Laue instruments and refining the DAXM technique for sub 200 nm resolution will pose significant technical challenges, particularly in terms of optics and long-term stability. Figure 4: Strain and lattice rotation. Estimated minimum and maximum strain and lattice rotation values for a misfit dislocation buried in the bulk. The vertical axes show direct strains ( a ) and shear strains ( b ) in units of micro strain (10 −6 ), and lattice rotations ( c ) in degrees. The horizontal axes show the probe FWHM in nm. In the strain and lattice rotation subscripts, x corresponds to the [IĪ0], y to the [00I] and z to the [ĪĪ0] direction. Superimposed in grey are the estimated experimental uncertainties. In b , the light grey area shows the anticipated uncertainty associated with the γ xy and γ yz (that is, γ –00I and γ 00I– ) shear strain components, whereas the dark grey area shows the uncertainty associated with the γ zx (that is, γ – ) component. The vertical dashed lines indicate the X-ray probe size used for the experiments reported here. Full size image In conclusion, we have demonstrated the first imaging of a single dislocation using micro-beam X-ray diffraction. The measurements were directly validated by TEM micrographs of the same dislocation, showing excellent agreement. Strains and lattice rotations determined by μ-Laue diffraction agree with those predicted by an anisotropically elastic model of the structure. Unlike TEM our method is not limited to thin, electron-transparent samples. Indeed our simulations indicate that 3D measurements of individual dislocations in the bulk should be feasible if sufficiently high spatial resolution DAXM approaches are developed. This work thus conclusively demonstrates that X-ray micro-diffraction techniques are now capable of characterizing materials at the single dislocation level. μ-Laue diffraction μ-Laue diffraction measurements were carried out at beamline 34-ID-E at the Advanced Photon Source (Argonne National Lab, IL, USA). The incident polychromatic X-ray beam (7–30 keV) was focussed by Kirkpatrick–Baez mirrors to a spot with near Lorentzian profile and FWHM of 0.6 μm vertically and 0.4 μm horizontally. Key parameters of the focussing arrangement on 34-ID-E are provided in Supplementary Table S1 . The GaAs/In 0.2 Ga 0.8 As/GaAs membrane was mounted in 45° reflection geometry with the dislocation line in the horizontal plane, perpendicular to the beam direction as illustrated in Fig. 1 and Supplementary Fig. S1 . Diffraction patterns were recorded on a Perkin-Elmer flat panel detector (409.6 × 409.6 mm 2 , 2,048 × 2,048 pixels, amorphous Si, CsI scintillator, 16-bit dynamic range corresponding to 65,536 counts) mounted in 90° reflection geometry 510.3 mm above the sample, spanning a solid angle of 0.56 steradians. The sample to detector distance was chosen as a compromise between minimizing strain measurement uncertainties due to geometrical perturbations [16] , capturing of a sufficient solid angle and number of Laue diffraction peaks (>30) for accurate strain refinement, and good peak position accuracy. Owing to its construction, image distortion of the Perkin-Elmer detector is minimal and does not need to be corrected for, unlike optical-taper-based CCD cameras. μ-Laue patterns were collected from a 40 × 60 μm 2 sample area, previously imaged with TEM, using a 0.5 μm step size and 1 s counting time. DAXM wire scans were not carried out as the available depth resolution of ~0.5 μm [20] was coarser than the membrane thickness of 129.5 nm. Data analysis was performed using the X-ray micro-diffraction analysis software (XMAS) [45] and LaueGo (J. Z. Tischler: tischler@anl.gov) software packages. Diffuse background scatter was removed using a median filtering approach [46] . Laue peaks were fitted in a 7 × 7 pixel window using a 2D Lorentzian function. In each Laue pattern, at least 40 peaks were indexed and used for strain refinement. Peak intensities ranged from 30 to 800 counts (corresponding to signal to noise ratios of 6–160) and each image contained at least 15 peaks with intensity >100 counts. Lattice rotations and strains were computed with respect to a nominally strain free reference, taken as their average value over the measurement region. Hence systematic offsets of lattice orientation and strain were removed. The specific alignment of the dislocation line ( Supplementary Fig. S1 ) was chosen to maximize the angular separation of Laue diffraction peaks from either side of the dislocation. In the chosen configuration, the 0.1° change in ω ĪĪ0 lattice orientation at the dislocation line caused a separation of Laue peaks by 0.2° due to alignment with the 2 θ direction. If the sample were rotated by 90° about its surface normal, peaks from either side of the dislocation would only be separated by 0.1°. From Fig. 2c it is clear that if the separation between peaks originating from either side of the dislocation were halved, significant overlap would make accurate fitting difficult. In terms of the measurable strain signal, the ability to separately index scattering contributions from either side of the dislocation line far outweighs the benefit of the improved spatial resolution had the sample been rotated by 90° about its surface normal. Simulation of dislocation strain fields in the membrane We considered a simulation plane perpendicular to the misfit dislocation line, that is, perpendicular to the [ĪĪ0] direction, as illustrated in Supplementary Fig. S2 . The solutions for an infinitely long dislocation in an elastically anisotropic medium with cubic symmetry [1] were superimposed with finite element calculations to solve the boundary value problem ( Supplementary Fig. S3 ). For the computation, the misfit dislocation with [ĪĪ0] line direction was split into three parts: an edge dislocation with burgers vector b IĪ0 =1.998 Å in the plane of the membrane, an edge dislocation with burgers vector b 00I =2.826 Å in the out-of-plane direction and a screw dislocation with burgers vector b ĪĪ0 =−1.998 Å, as illustrated in Supplementary Fig. S2(b) . Calculations for the three cases were carried out separately and then summed to give the overall displacement, strain and lattice rotation fields. Anisotropic elastic constants for GaAs from the literature were used ( C 11 =119.0 GPa, C 12 =53.8 GPa and C 44 =59.5 GPa) [37] . Finite element calculations were carried out using the CAST3M code ( http://www-cast3m.cea.fr ), whereas the remainder of the computation was carried out in Matlab. Plots of the resulting deviatoric strain, stress and lattice rotation fields are shown in Supplementary Figs S4–S6 , respectively. Interestingly, although GaAs has significant elastic anisotropy, a comparison with calculations assuming GaAs to be elastically isotropic ( Supplementary Figs S7–S9 ) shows little difference between the isotropic and anisotropic models. To calculate the anticipated strain and rotation profiles for comparison with the experimental data, a convolution approach was used, in which the X-ray beam is represented by a probe sensitivity function and scattering contributions form either side of the dislocation line are treated separately. Further details of these simulations are provided in Supplementary Notes 2 and 3 . How to cite this article: Hofmann, F. et al. X-ray micro-beam characterization of lattice rotations and distortions due to an individual dislocation. Nat. Commun. 4:2774 doi: 10.1038/ncomms3774 (2013).